Single-shot three-dimensional structure determination of nanocrystals with femtosecond X-ray free-electron laser pulses Conventional three-dimensional (3D) structure determination methods require either multiple measurements at different sample orientations or a collection of serial sections through a sample. Here we report the experimental demonstration of single-shot 3D structure determination of an object; in this case, individual gold nanocrystals at ~5.5 nm resolution using ~10 fs X-ray free-electron laser pulses. Coherent diffraction patterns are collected from high-index-faceted nanocrystals, each struck by an X-ray free-electron laser pulse. Taking advantage of the symmetry of the nanocrystal and the curvature of the Ewald sphere, we reconstruct the 3D structure of each nanocrystal from a single-shot diffraction pattern. By averaging a sufficient number of identical nanocrystals, this method may be used to determine the 3D structure of nanocrystals at atomic resolution. As symmetry exists in many virus particles, this method may also be applied to 3D structure studies of such particles at nanometer resolution on femtosecond time scales. Coherent diffraction imaging (CDI) using synchrotron radiation [1] , [2] , [3] , [4] , [5] , [6] , [7] , [8] , [9] , [10] , [11] , [12] , [13] , X-ray free-electron lasers (XFELs) [14] , [15] , [16] , [17] , high harmonic generation [18] , [19] , [20] , [21] , soft X-ray lasers [19] , [22] , [23] , optical lasers [24] , [25] , [26] and electrons [27] is a rapidly growing area of research that has found applications across several disciplines. One of the major potential applications of CDI is to determine the three-dimensional (3D) structure of single particles at atomic resolution on few-femtosecond timescales [28] , [29] , [30] , [31] . Recent experiments have confirmed that the two-dimensional (2D) diffraction pattern of a single particle can be recorded and reconstructed from a single XFEL pulse before the onset of radiation damage [14] , [15] , [17] . However, although a method termed ankylography was recently proposed to obtain 3D structure from a single sample orientation [22] , single-shot 3D imaging has not been experimentally realized as yet. In this article, we perform single-shot 3D structure determination of high-index-faceted gold nanocrystals. Nanocrystals are widely used in modern science and technology owing to their physical and chemical properties that can be engineered in ways that are very different from either molecules or bulk solids [32] . The optical, catalytic, electronic and magnetic properties of nanocrystals are strongly related to their shape, size and structure [32] . Conventional methods used to characterize nanocrystals include transmission electron microscopy (TEM), scanning electron microscopy (SEM), electron tomography, atomic force microscopy (AFM), X-ray and electron diffraction [32] , [33] , [34] , [35] , [36] . Here we demonstrate single-shot 3D structure determination of large (~100 nm) and catalytically active nanocrystals using single ~10 fs XFEL pulses. Coherent diffraction patterns are collected from high-index-faceted gold nanocrystals, each struck by a single XFEL pulse based on the diffraction-before-destruction scheme [14] , [15] , [17] . Using the symmetry of the nanocrystals and the curvature of the Ewald sphere [22] , we reconstruct the 3D structure of each nanocrystal from a single-shot diffraction pattern to determine the high-index {661} facets with ~5.5 nm resolution on ~10 fs timescales. Furthermore, the single-shot diffraction patterns of identical nanocrystals were selected to assemble a 3D diffraction pattern, from which an average 3D reconstruction was achieved with a resolution presently limited by the detector geometry. Single-shot XFEL experiment The experiment was conducted using the SPring-8 Angstrom Compact Free-Electron Laser (SACLA) [37] . 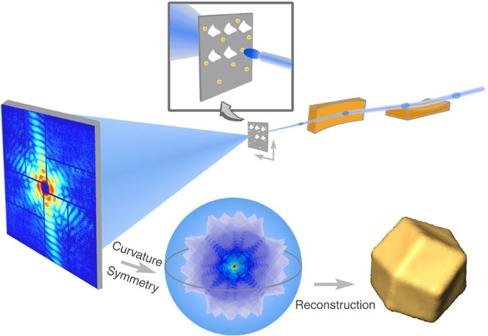Figure 1: Schematic layout of the single-shot 3D structure determination using femtosecond XFEL pulses. XFEL pulses were focused to a ~1.5-μm spot by a pair of K-B mirrors. Single-shot diffraction patterns were acquired from high-index-faceted gold nanocrystals based on the diffraction-before-destruction scheme. By using the symmetry of the nanocrystal and the curvature of the Ewald sphere, a 3D diffraction pattern was generated from a single-shot diffraction pattern, from which a 3D reconstruction was computed with a resolution of ~5.5 nm. Figure 1 shows a schematic layout of the experimental setup. XFEL pulses (photon energy: 5.4 keV, pulse duration: ~10 fs, and pulse energy at the source: ~300 μJ) were focused to a ~1.5-μm spot by a pair of Kirkpatrick-Baez (K-B) mirrors [38] , [39] . The focused XFEL pulses impinged on high-index-faceted gold nanocrystals deposited on a 100-nm-thick Si 3 N 4 membrane. The gold nanocrystals, synthesized by the seed-mediated growth method to ensure monodisperse trisoctahedral shape and size (see Methods), consist of a high density of low-coordinated atoms such as steps, edges and kinks, serving as catalytically active sites [40] , [41] . By scanning the Si 3 N 4 membrane relative to the focused XFEL pulses, coherent X-ray diffraction patterns were collected on a multi-port charge coupled device (CCD) detector, each generated from a randomly orientated nanocrystal with a single pulse (see Methods) [42] , [43] . Supplementary Movie 1 shows a typical single-shot XFEL experiment. The density of nanocrystals deposited on the Si 3 N 4 membrane was tuned to control the hit-rate for these experiments. Supplementary Fig. 1 shows the nanocrystals deposited on a Si 3 N 4 membrane before and after being struck by XFEL pulses. Using this data acquisition scheme, we collected a total of 126,976 X-ray diffraction patterns, including no hits, partial hits, single-particle hits and multiple-particle hits. After screening and post analysis (see Methods), we obtained 1,877 diffraction patterns with single-particle hits and a hit rate of ~2.3%, from which 100 good quality diffraction patterns were selected from single isolated and highly symmetrical nanocrystals ( Supplementary Movie 2 ). The best six single-shot diffraction patterns are shown in Fig. 2a and Supplementary Fig. 2 , whose diffraction signal is presently limited by the detector geometry employed. Figure 1: Schematic layout of the single-shot 3D structure determination using femtosecond XFEL pulses. XFEL pulses were focused to a ~1.5-μm spot by a pair of K-B mirrors. Single-shot diffraction patterns were acquired from high-index-faceted gold nanocrystals based on the diffraction-before-destruction scheme. By using the symmetry of the nanocrystal and the curvature of the Ewald sphere, a 3D diffraction pattern was generated from a single-shot diffraction pattern, from which a 3D reconstruction was computed with a resolution of ~5.5 nm. 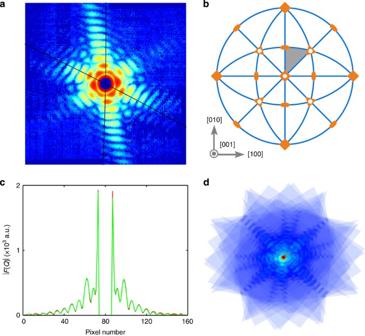Figure 2: Symmetry verification of the trisoctahedral gold nanocrystals using the self-common arcs present in each single-shot diffraction pattern. (a) A representative single-shot diffraction pattern, where 13 × 13 pixel binning of the highly oversampled intensity makes the narrow missing bars of the detector essentially disappear. (b) Stereographic projection of trisoctahedral symmetry, belonging to crystallographic point groupand consisting of two- (ellipsis symbols), three- (triangle symbols), fourfold (diamond symbols) rotational symmetry and the centro-symmetry (white circles). (c) A representative pair of self-common arcs, corresponding to two dark curves ina. (d) After verifying the trisoctahedral symmetry, a 3D diffraction pattern was assembled from 48 symmetrized copies of the single-shot diffraction pattern (a). Full size image Figure 2: Symmetry verification of the trisoctahedral gold nanocrystals using the self-common arcs present in each single-shot diffraction pattern. ( a ) A representative single-shot diffraction pattern, where 13 × 13 pixel binning of the highly oversampled intensity makes the narrow missing bars of the detector essentially disappear. ( b ) Stereographic projection of trisoctahedral symmetry, belonging to crystallographic point group and consisting of two- (ellipsis symbols), three- (triangle symbols), fourfold (diamond symbols) rotational symmetry and the centro-symmetry (white circles). ( c ) A representative pair of self-common arcs, corresponding to two dark curves in a . ( d ) After verifying the trisoctahedral symmetry, a 3D diffraction pattern was assembled from 48 symmetrized copies of the single-shot diffraction pattern ( a ). Full size image Symmetry verification of the single-shot diffraction patterns Trisoctahedral nanocrystals belong to the crystallographic point group , consisting of two-, three- and fourfold rotational symmetry along the <011>, <111> and <001> directions, respectively ( Fig. 2b ). Given a single-shot diffraction pattern of a trisoctahedral nanocrystal sampled on the Ewald sphere, there are 48 symmetry operations that can generate 48 spherical diffraction patterns. These diffraction patterns intersect with each other to form 14 independent pairs of self-common arcs (see Methods). By analyzing the six single-shot diffraction patterns, we confirmed the existence of 14 independent pairs of self-common arcs in each diffraction pattern. Figure 2c and Supplementary Fig. 3 show four representative pairs of the self-common arcs for Fig. 2a . We quantified the self-common arcs for the six single-shot diffraction patterns by using R arc (see Methods). The average R arc for the six diffraction patterns is 5.8, 6.9, 8.4, 8.8, 9.1 and 9.5%. The small R arc values suggest that these single-shot diffraction patterns have high signal-to-noise ratios, and that our screening and post data analysis approach allows us to select single-shot diffraction patterns from highly symmetrical nanocrystals. 3D phase retrieval with symmetry After verifying the trisoctahedral symmetry of the nanocrystals, the orientation of each single-shot diffraction pattern was determined, from which a 3D diffraction pattern was generated using symmetry ( Fig. 2d; see Methods). The 3D diffraction pattern was then iteratively phased to obtain a high-resolution image by incorporating symmetry into the oversampling smoothness (OSS) algorithm [44] . For each 3D diffraction pattern, we first performed 100 independent OSS reconstructions with random phases as their initial input, each consisting of 2,000 iterations and using a box as a loose support. For each independent reconstruction, symmetry was used as a constraint in real space and enforced once every 30 iterations (see Methods). By averaging the five best reconstructions, we determined a tight support and performed another 100 independent OSS reconstructions, again enforcing symmetry once every 30 iterations. The five best reconstructions were averaged to obtain a final 3D image. 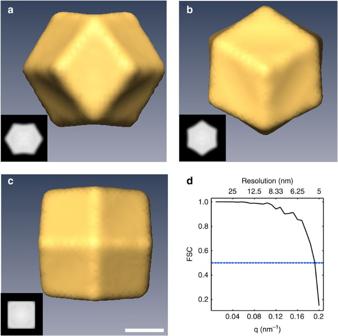Figure 3: 3D reconstruction of the single-shot diffraction pattern (Fig. 2a). (a–c) Iso-surface renderings of the final 3D reconstruction along the two-, three- and fourfold rotational symmetry, respectively (a threshold of 30% of the maximum density was used to display these images). The insets show 3.3-nm-thick centro-slices of the 3D reconstruction along the corresponding directions. The variation of the electron density inside the nanocrystal is within ±10%, which is mainly due to noise in the single-shot diffraction pattern and the intensity variation inside each XFEL pulse. (d) FSC comparison between two independently reconstructed gold nanocrystals. Based on the FSC=0.5 criterion, a 3D resolution of the reconstructions was estimated to be ~5.5 nm. The iso-surface rendering images as well as those inFigs 4and6are displayed by Amira with interpolation. Scale bar, 30 nm. Figure 3a–c , and Supplementary Movie 3a show iso-surface renderings of the final image along the two-, three- and fourfold rotational symmetry, reconstructed from Fig. 2a . The concave facets of the nanocrystal are visible, and the insets show three 3.3-nm-thick centro-slices of the image. Using the same procedure, we obtained final 3D reconstructions from five other single-shot diffraction patterns ( Supplementary Fig. 4 ). To investigate whether enforcing symmetry in the phase retrieval algorithm influenced the shape and structure of the reconstructed nanocrystals, we conducted numerical simulations on single-shot 3D structure determination of cubic, octahedral and trisoctahedral nanocrystals ( Supplementary Fig. 5 ), all belonging to the point group (see Methods). Using simulated single-shot diffraction patterns ( Supplementary Fig. 6 ) at random orientations, we applied the same procedures to first determine the orientation of each diffraction pattern and then achieve a single-shot 3D reconstruction. Supplementary Fig. 7 shows the 3D reconstructions of the cubic, octahedral and trisoctahedral nanocrystals, which are in good agreement with the 3D models ( Supplementary Fig. 5 ). These results indicate that the shape, size and facets of the 3D reconstructions are intrinsically encoded in the single-shot diffraction patterns. Figure 3: 3D reconstruction of the single-shot diffraction pattern ( Fig. 2a ). ( a – c ) Iso-surface renderings of the final 3D reconstruction along the two-, three- and fourfold rotational symmetry, respectively (a threshold of 30% of the maximum density was used to display these images). The insets show 3.3-nm-thick centro-slices of the 3D reconstruction along the corresponding directions. The variation of the electron density inside the nanocrystal is within ±10%, which is mainly due to noise in the single-shot diffraction pattern and the intensity variation inside each XFEL pulse. ( d ) FSC comparison between two independently reconstructed gold nanocrystals. Based on the FSC=0.5 criterion, a 3D resolution of the reconstructions was estimated to be ~5.5 nm. The iso-surface rendering images as well as those in Figs 4 and 6 are displayed by Amira with interpolation. Scale bar, 30 nm. Full size image 3D resolution estimation and structure quantification To evaluate the resolution of the six single-shot 3D reconstructions, we calculated the Fourier shell correlation (FSC) between the independent reconstructions of the six nanocrystals (see Methods) [45] , [46] . Figure 2c and Supplementary Fig. 8 show four representative FSC curves. Based on the FSC=0.5 criterion, which has been widely used to estimate the resolution in single-particle cryo-electron microscopy (EM) [45] , [46] , [47] , we estimated the 3D resolution of these reconstructions to be ~5.5 nm. Next, we quantified the structure, shape and size of these reconstructed gold nanocrystals. 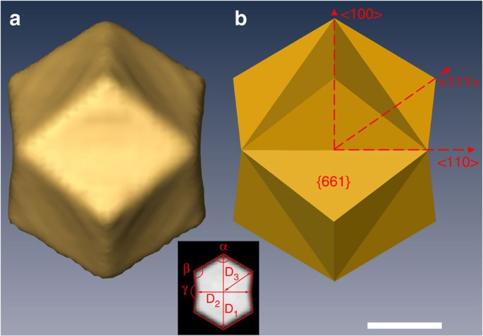Figure 4: 3D model of a trisoctahedral gold nanocrystal constructed from a single-shot 3D reconstruction. (a) Iso-surface rendering and 3.3-nm-thick central slice (inset) of the nanocrystal along the twofold rotational symmetry reconstructed fromFig. 2a, of whichD1,D2,D3,α,βandγare six parameters used to characterize the shape, size and facets of the nanocrystal. (b) 3D model of the concave trisoctahedral nanocrystal constructed froma, containing exposed high index {661} facets (see Methods). Scale bar, 30 nm. Figure 4a and the inset show an iso-surface rendering and a 3.3-nm-thick central slice of a representative reconstructed nanocrystal along the twofold rotational symmetry, for which D 1 , D 2 , D 3 , α , β and γ are six parameters used to characterize the shape, size and facets of the nanocrystal. For each nanocrystal, we first determined the 3D orientations of the 24 facets and then measured the six parameters ( Table 1 ). To quantify these measurements, we calculated the mean and standard deviation of D 1 , D 2 , D 3 , α , β and γ to be 102.3±0.5 nm, 72.3±0.4 nm, 48.5±0.3 nm, 119.3±0.5°, 113.4±0.5° and 166.1±0.6°, respectively, for the six nanocrystals. The consistency of these values indicates that their overall shape and size are in good agreement. The three interfacial angles ( α , β and γ ) measured from all six nanocrystals agree with the values expected for a concave trisoctahedron with exposed {661} index facets (see Methods and Table 1 ). To further verify the {661} index facets, we calculated the interfacial angles of possible { hhl } index facets for a trisoctahedron ( Supplementary Table 1 ), indicating that there are at least 1.4°, 1.7° and 1.9° differences for angles α , β and γ between {661} and other facets. As our six independent measurements of the three interfacial angles are more accurate than these angular differences ( Table 1 ), this further confirms that the concave trisoctahedral gold nanocrystals contain exposed high-index {661} facets ( Fig. 4b ). Finally, TEM, SEM and AFM images were taken from the similar gold nanocrystals to verify their exposed high-index facets ( Supplementary Figs 9–11 ). Figure 4: 3D model of a trisoctahedral gold nanocrystal constructed from a single-shot 3D reconstruction. ( a ) Iso-surface rendering and 3.3-nm-thick central slice (inset) of the nanocrystal along the twofold rotational symmetry reconstructed from Fig. 2a , of which D 1 , D 2 , D 3 , α , β and γ are six parameters used to characterize the shape, size and facets of the nanocrystal. ( b ) 3D model of the concave trisoctahedral nanocrystal constructed from a , containing exposed high index {661} facets (see Methods). Scale bar, 30 nm. Full size image Table 1 Six parameters ( D 1 , D 2 , D 3 , α , β and γ ), used to characterize the shape, size and facets of the trisoctahedral nanocrystals, were measured for seven independent reconstructions. Full size table 3D reconstruction of the average structure of the nanocrystals After achieving single-shot 3D structure determination of the nanocrystals, we conducted 3D reconstruction of the average structure from six single-shot diffraction patterns. Cross-common arcs were used to examine whether the diffraction patterns were generated from identical gold nanocrystals. Thirty pairs of cross-common arcs exist between six spherical diffraction patterns (see Methods). 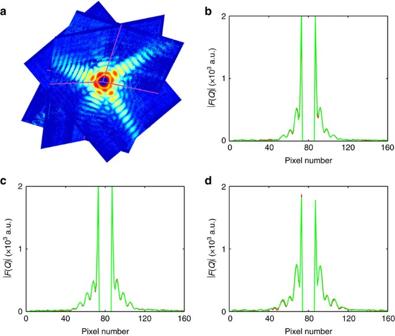Figure 5: Cross-common arcs used to align different single-shot diffraction patterns. (a) Three single-shot diffraction patterns form six pairs of cross-common arcs. (b–d) Three representative pairs of the cross-common arcs between the three diffraction patterns shown ina. Figure 5 shows three representative pairs of the cross-common arcs between three single-shot diffraction patterns. The average R arc of the 30 pairs of cross-common arcs was calculated to be 9.7%, which is comparable to those obtained from the self-common arcs. After determining the relative orientations of the six single-shot patterns, we assembled a 3D diffraction pattern from 288 symmetrized 2D diffraction patterns (48 for each of the six nanocrystals). Using OSS with symmetry (see Methods), we reconstructed the average 3D structure of the gold nanocrystals ( Fig. 6 , and Supplementary Movie 3b ). The six parameters ( D 1 , D 2 , D 3 , α , β and γ ) measured for the average structure are very consistent with a concave trisoctahedral nanocrystal containing exposed high-index {661} facets ( Table 1 ). We also quantified the average 3D structure with respect to the single-shot 3D reconstructions by calculating FSC curves between them ( Supplementary Fig. 12 ), indicating that the resolution of the average 3D reconstruction is presently limited by the detector geometry used. Figure 5: Cross-common arcs used to align different single-shot diffraction patterns. ( a ) Three single-shot diffraction patterns form six pairs of cross-common arcs. ( b – d ) Three representative pairs of the cross-common arcs between the three diffraction patterns shown in a . 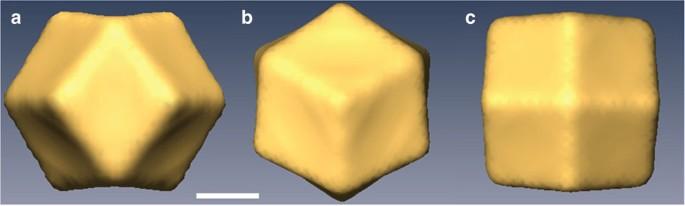Figure 6: 3D reconstruction of the average structure of the nanocrystals. (a–c) Iso-surface renderings of the average trisoctahedral nanocrystal along the two-, three- and fourfold symmetry, respectively, reconstructed from a 3D diffraction pattern assembled from 288 symmetrized 2D patterns (48 for each single-shot diffraction pattern). Scale bar, 30 nm. Full size image Figure 6: 3D reconstruction of the average structure of the nanocrystals. ( a – c ) Iso-surface renderings of the average trisoctahedral nanocrystal along the two-, three- and fourfold symmetry, respectively, reconstructed from a 3D diffraction pattern assembled from 288 symmetrized 2D patterns (48 for each single-shot diffraction pattern). Scale bar, 30 nm. Full size image Although symmetry has long been used to determine the 3D structures of virus particles with EM [48] , [49] , this work represents the first combination of symmetry and CDI for achieving single-shot 3D structure determination of nanocrystals at ~5.5 nm resolution using ~10 fs XFEL pulses. The significance of the present work is threefold. First (to our knowledge), a 3D resolution of ~5.5 nm is the highest resolution ever achieved in any 3D X-ray imaging method. Second, as symmetry exists in many nanocrystals and virus particles [32] , [40] , [41] , [48] , [49] , [50] , this method may be applied to 3D structure studies of such particles at nanometer resolution on femtosecond timescales. For the virus particles, symmetry exists in the capsid, but not in the internal DNA or RNA genome [48] , [49] , [50] . Thus, the method can only be used to determine the 3D structure of the capsid but not the internal genome of the virus particles. Third, the intense, femtosecond XFEL pulses allow us to select single-shot diffraction patterns from highly symmetrical and identical nanocrystals based on self- and cross-common arcs (see Methods). With a sufficient number of identical nanocrystals, this approach may be used to determine the 3D structure of nanocrystals at atomic resolution. Compared with TEM, electron diffraction and electron tomography that achieve higher resolutions [33] , [34] , [35] , [36] , [51] , this imaging technique can study thicker nanocrystals with negligible dynamic scattering effects. Thus, we expect this work may find applications in CDI, XFEL science, materials science, nanoscience, chemistry and structural biology. Synthesis of monodisperse trisoctahedral gold nanocrystals Monodisperse trisoctahedral gold nanocrystals were synthesized by a seed-mediated growth method using cetyltrimethylammonium chloride as the capping agent [40] , [41] . First, the gold seeds with a diameter of ~3.5 nm were prepared. Then by adding the gold seed solution into the cetyltrimethylammonium chloride growth solution, better control of the gold atom concentration in the solution was achieved, thereby allowing the growth kinetics of the gold nanocrystals to be manipulated and preservation of their concave trisoctahedral shape while the nanocrystals grew synchronously in size. The size of gold nanocrystals was controlled by adjusting the number of additional seeds. The synthesized trisoctahedral gold nanocrystals were examined by TEM, SEM and AFM, indicating their size variation is within 5% except for few special cases ( Supplementary Figs 9–11 ). Data acquisition The single-shot XFEL experiment was conducted using the multiple application X-ray imaging chamber (MAXIC) installed in experimental hutch 3 of SACLA [42] . Gold nanocrystals, positioned randomly on a 100-nm-thick Si 3 N 4 membrane, were exposed to single XFEL pulses with wavelength of ~2.3 Å. The pulse energy was measured to be ~300 μJ at the source and ~100 μJ at the sample. The single-shot exposures were automated using a 2D scan programme that controlled both the XFEL pulse selector and the sample motor stage, ensuring only a single XFEL pulse impinged on the Si 3 N 4 membrane at a programmed position. The sample was destroyed after exposure to a single XFEL pulse, leaving a hole in the membrane ( Supplementary Fig. 1 ). Although the XFEL pulses are delivered at a repetition rate of 10 Hz, the single-shot exposures can be performed at either 1 or 10 Hz. The present experiment was performed at 1 Hz. The single-shot X-ray diffraction patterns were recorded by an octal sensor, multiport CCD (octal-MPCCD) detector with 2,048 × 2,048 pixels and a pixel size of 50 × 50 μm (ref. 43 ). The octal-MPCCD was designed to allow an adjustable central aperture varying from complete closure to a maximum opening of 10 × 10 mm 2 . The detector was placed at 1.47 m downstream of the sample, and the central aperture was set at 3 × 3 mm 2 . The parasitic scatterings from the K-B mirrors as well as other X-ray optics were blocked by two sets of four-way cross slits inside the MAXIC; one set positioned close to the sample (at a distance of ~20 mm) and the other set further upstream of the sample (at a distance of ~350 mm). The experiment was performed under a vacuum pressure of ~10 −4 Pa within the MAXIC chamber. Data screening and post analysis Using the data acquisition scheme described above, we have collected 126,976 diffraction patterns. To detect ‘true hits’ within the collected data, we employed a data screening approach by comparing the average intensity in a pre-defined region of the detector with a threshold. By examining different thresholds heuristically, we were able to differentiate between no hits, partial hits, exact single-particle hits and multiple-particle hits. After data screening, we obtained 2,877 single-particle hits (corresponding to a hit rate of ~2.3%), from which 100 single-shot diffraction patterns were selected for further analysis ( Supplementary Movie 2 ). We then performed background subtraction to remove the detector read-out noise, located the centre for each of the 100 diffraction patterns and performed 13 × 13 pixel binning of the diffraction intensity (see Methods) [52] . Next, we applied a curvature correction to the diffraction patterns (see Methods). Although the effect of the curvature of the Ewald sphere is small, it is not negligible in this experiment. The diffraction intensity extended to a highest resolution of ~4.6 nm, corresponding to a maximum diffraction angle (2 θ max ) of 2.87°, which was limited by the detector geometry used. As each 2D diffraction pattern was collected by a planar CCD detector, we projected the diffraction intensity onto the Ewald sphere by re-sampling the intensity points (see Methods) [22] . After the curvature correction, we prioritized the 100 single-shot diffraction patterns by evaluating the self-common arcs and calculating an average R arc for each diffraction pattern (see Methods). The six single-shot diffraction patterns ( Fig. 2a and Supplementary Fig. 2 ) with the smallest R arc were chosen for further analysis and reconstructions. 13 × 13 Pixel binning for each single-shot diffraction pattern The single-shot diffraction patterns were measured by an octal-MPCCD, which includes several missing bars with a bar width ranging from 2 to 8 pixels ( Fig. 1 ). To remove the missing bars and enhance the signal-to-noise ratio of the diffraction patterns, we performed 13 × 13 pixel binning of the diffraction intensity [52] . If more than 50% of the 13 × 13 pixels were measured, the pixel after binning was set to be the average value of the measured pixels. Otherwise, the pixel after binning was set to be a missing pixel. The linear oversampling ratio before binning is between 67 and 94 (depending on the orientation of the nanocrystal) and becomes between 5 and 7 after binning [53] , [54] . Because of the large oversampling ratio, the binning process makes the narrow missing bars of the detector essentially disappear ( Fig. 2a ). Curvature correction of the single-shot diffraction patterns As each single-shot diffraction pattern was measured by a planar CCD detector, the solid angle subtended by each pixel is not a constant. The increase of the spatial frequency of the diffraction intensity corresponds to the decrease of the solid angle subtended by each pixel. We normalized the diffraction intensity by [22] where and are the normalized and measured diffraction intensities, Ω 0 and are the solid angle subtended by the centro-pixel and pixel , respectively. After intensity normalization, we projected each single-shot diffraction pattern onto the surface of the Ewald sphere, which was then interpolated to assemble a 3D diffraction pattern by using symmetry (see Methods). Self-common arcs in single-shot diffraction patterns The trisoctahedral symmetry belongs to the crystallographic point group , consisting of 48 symmetry operations [55] . The shaded area in Fig. 2b shows the fundamental domain of a trisoctahedron, from which all the other 47 domains can be generated by symmetry operations. Using symmetry, each 2D diffraction pattern sampled on the Ewald sphere can produce a total of 48 symmetrized copies. The 48 symmetrized diffraction patterns form 47 common arcs (instead of common lines as in single particle EM [48] , [49] ), which we term self-common arcs. After mathematically examining each of the 47 pairs of self-common arcs, we found that 14 of them are independent and the other 33 pairs are either redundant or exactly identical. Next, we verified the trisoctahedral symmetry of the gold nanocrystals based on the 14 pairs of independent self-common arcs. For each single-shot diffraction pattern, we searched for the 14 pairs of self common arcs with 0.5° per step along each of the three Euler angles ( φ , θ , ω ) in the fundamental domain. Each pairs of independent self-common arcs are quantified by where and represent the Fourier modulus on arcs 1 and 2, respectively. We calculated an average R arc from the 14 individual R arc values. By scanning all the angles in the fundamental domain, we found a global minimum of the average R arc for each single-shot diffraction pattern, confirming the existence of the trisoctahedral symmetry in the diffraction pattern. The six single-shot diffraction patterns with the smallest average R arc were chosen from the 100 patterns. The average R arc for the six selected diffraction patterns is 5.8, 6.9, 8.4, 8.8, 9.1 and 9.5%. Figure 2c and Supplementary Fig. 3b–d show four representative self-common arcs for the diffraction pattern of Fig. 2a . The small R arc values indicate that these single-shot diffraction patterns have high signal-to-noise ratios and were generated from highly symmetrical trisoctahedral nanocrystals. Cross-common arcs between single-shot diffraction patterns To examine whether the single-shot diffraction patterns were generated from identical trisoctahedral gold nanocrystals, we calculated the common arcs between different diffraction patterns (termed cross-common arcs) [49] , [56] , [57] . For six single-shot diffraction patterns sampled on the Ewald sphere, there are 30 pairs of cross-common arcs (there would be 15 pairs of cross-common lines if the diffraction patterns are sampled on a plane). By performing 3D searching of the cross-common arcs with 0.5° per step along each of the three Euler angles ( φ , θ , ω ) in the fundamental domain, we found the 30 pairs of cross-common arcs between the six single-shot diffraction patterns. Supplementary Fig. 12b–d shows three representative pairs of cross-common arcs. We also calculated an average R arc for the 30 pairs of cross-common arcs to be 9.7%, which is comparable to those obtained from the self-common arcs. Generating 3D diffraction patterns via symmetry Based on the self- and cross-common arcs for the six single-shot diffraction patterns (see Methods), we determined the orientation of each diffraction pattern with respect to a set of symmetry-related primary axes ( Fig. 2b ). Using the symmetry operations, a 3D diffraction matrix on a Cartesian grid was generated from 48 symmetrized diffraction patterns. The value of a Cartesian point was calculated through linear interpolation of the neighbouring points available from the symmetrized Fourier modulus (that is, the square root of the diffraction intensity). Specifically, we assigned each Cartesian point at the origin of a sphere with a radius of 0.4 voxels, for which we defined the measured points within the sphere. We then interpolated the value of the Cartesian grid by where and are the Fourier modulus of Cartesian grid and measured point , N is the total measured points within the sphere and is the distance between points and . If N =0, we assigned the value of the corresponding Cartesian point undefined. This 3D interpolation approach yielded seven 3D diffraction patterns, six of which were obtained from the individual single-shot diffraction patterns and the seventh was assembled by combining the six patterns. Incorporation of symmetry into the OSS algorithm After verifying the existence of trisoctahedral symmetry in the single-shot diffraction patterns based on self-common arcs (see Methods), we incorporated the symmetry constraint into the OSS algorithm [44] . As the point group is Fourier transform invariant, no interpolation is needed to enforce the symmetry operations during the phase retrieval process. To implement the symmetry constraint, we first located the voxels in the fundamental domain in real space. We then applied the symmetry operations to these voxels to find the corresponding voxels in the other 47 domains. We averaged the symmetry-related voxels in the 48 domains and assign each voxel the averaged value. For each 3D diffraction pattern, we performed 100 independent OSS reconstructions with a box as a loose support, where each reconstruction consisted of 2,000 iterations and the symmetry constraint was enforced once every 30 iterations. The figure of merit for each reconstruction was monitored by an R f , defined as the difference between the experimental Fourier modulus and the calculated Fourier modulus in each iteration [44] . From each set of 100 reconstructions, we averaged the best five reconstructions with the smallest R f , from which we determined a tight support. Using this improved support, we performed another set of 100 independent OSS reconstructions for each 3D diffraction pattern under the same procedure as the loose support case. The best five reconstructions were averaged to obtain the final 3D image for each diffraction pattern. Numerical simulations on single-shot 3D structure determination We have performed numerical simulations to verify the feasibility of achieving 3D structure determination from a single-shot diffraction pattern. First, we simulated XFEL pulses with the same photon energy and pulse fluence as the experimental case in which the intensity variation within each XFEL pulse was not considered in the simulations. The XFEL pulses impinged on ~100 nm individual nanocrystals consisting of cubic, octahedral and trisoctahedral shapes ( Supplementary Fig. 5 ), which belong to the same crystallographic point group (ref. 55 ). Next, we generated a single-shot diffraction pattern from each of the cubic, octahedral and trisoctahedral nanocrystals with three random Euler angles ( φ , θ , ω ). We then added Poisson noise to the diffraction patterns and removed the low spatial frequency intensity to simulate a beam stop. Each simulated single-shot diffraction pattern ( Supplementary Fig. 6 ) looks similar to the experimental one ( Fig. 2a and Supplementary Fig. 2 ). For each diffraction pattern, we searched for the 14 self-common arcs (see Methods) from which its orientation, that is, the three Euler angles ( φ , θ , ω ), was determined. After orientation determination, a 3D diffraction pattern was assembled from the single-shot pattern based on the symmetry and the curvature of the Ewald sphere (see Methods). The phase retrieval of the 3D diffraction pattern was performed by incorporation of symmetry into the OSS algorithm (see Methods). Supplementary Fig. 7 shows the 3D reconstruction of the cubic, octahedral and trisoctahedral nanocrystals from single-shot diffraction patterns, which are in good agreement with the original structures ( Supplementary Fig. 5 ). Resolution estimation based on the FSC FSC has been widely used to estimate the 3D resolution in single-particle imaging with cryo-EM [45] , [46] , [47] . In this experiment, we determined the resolution based on the FSC method. First, we calculated 15 FSC curves between six independent single-shot 3D reconstructions. Supplementary Fig. 8 shows four representative FSC curves. Presently, there are two ways to estimate the resolution based on the FSC curves [46] , [47] : one with FSC=0.143 and the other with FSC=0.5. In our experiment, we adopted a more conservative criterion (FSC=0.5) to evaluate the resolution. Based on the 15 independent FSC curves, we determined the resolution of the single-shot 3D reconstructions to be consistently ~5.5 nm. Next, we calculated six FSC curves between the single-shot reconstructions and the average 3D reconstruction. Supplementary Fig. 12 shows four representative FSC curves, indicating that the resolution (~5.5 nm) of the 3D reconstruction of the assembled pattern is presently limited by the detector geometry used. Verification of the {661} index facets for the gold nanocrystals According to the crystallographic point group , the three interfacial angles ( α , β and γ ) for a concave trisoctahedron with { hhl } index facets is determined by [40] , [55] , The three interfacial angles calculated from Equation (4) for {661} index facets are 119.0°, 113.8° and 166.6°, which are consistent with the measured values ( Table 1 ). Compared with the estimation of the interfacial angles using 2D TEM images [40] , [41] , our measurements are based on the 3D facets and are intrinsically more accurate. To further verify the index facets and our model, we calculated the three interfacial angles for a concave trisoctahedron with possible { hhl } index facets ( Supplementary Table 1 ). These results indicate that there are at least 1.4°, 1.7° and 1.9° differences for angles α , β and γ between {661} facets and other index facets. As our six independent measurements of the three interfacial angles ( Table 1 ) are more accurate than these angular differences, this further confirms that the trisoctahedral gold nanocrystals contain {661} index facets. How to cite this article: Xu, R. et al. Single-shot three-dimensional structure determination of nanocrystals with femtosecond X-ray free-electron laser pulses. Nat. Commun. 5:4061 doi: 10.1038/ncomms5061 (2014).